Crystal growth within a phase change memory cell In spite of the prominent role played by phase change materials in information technology, a detailed understanding of the central property of such materials, namely the phase change mechanism, is still lacking mostly because of difficulties associated with experimental measurements. Here, we measure the crystal growth velocity of a phase change material at both the nanometre length and the nanosecond timescale using phase-change memory cells. The material is studied in the technologically relevant melt-quenched phase and directly in the environment in which the phase change material is going to be used in the application. We present a consistent description of the temperature dependence of the crystal growth velocity in the glass and the super-cooled liquid up to the melting temperature. Chalcogenide materials undergoing reversible crystal-to-amorphous phase transition continue to play a key role in information technology. In particular, phase change memory (PCM) has recently emerged as the most promising new nonvolatile solid-state memory technology [1] , [2] , [3] . Phase-change materials are also being investigated as building blocks of neuromorphic computing hardware [4] , [5] , [6] . A key property that makes these materials attractive for applications is the crystallization process that occurs at the nanometre length scale [7] and the nanosecond timescale [8] . Moreover, in spite of this fast crystallization rate at elevated temperatures, the melt-quenched amorphous state at lower temperatures is stable for several years [9] . Investigations of this unique crystallization process are being pursued using ab initio molecular dynamics simulations by several groups [10] , [11] , [12] . However, given the length and timescale associated with the crystallization process, experimental measurements are extremely challenging. At the technologically relevant nanometre length scale and nanosecond timescale, nucleation is expected to become less important and crystallization will be mostly governed by crystal growth. This is particularly true in the melt-quenched amorphous state, where already a large population of nuclei exists and a crystal/amorphous interface is present [13] . Most experimental investigations on the crystal growth velocity have been limited to low temperatures, where the crystallization rate is small. A recent effort to measure the growth rate is that by Orava et al. [14] , who used ultrafast differential scanning calorimetry. These measurements were conducted on as-deposited phase change materials. A more recent effort used laser-based time-resolved reflectivity measurements [15] . Despite pushing up the temperature range over which the crystallization rate was measured, both techniques were limited to temperatures below the temperature of the maximum growth velocity and far below the melting temperature. A widely accepted model describing the temperature dependence of crystal growth is [15] where r atom is the atomic radius, λ is the diffusional jump distance, R hyd is the hydrodynamic radius and k B denotes the Boltzmann constant. The term in the square brackets captures the thermally activated atomic transfer across the solid–liquid interface. Δ G ( T ) is the Gibbs energy difference between the liquid and the crystalline phase and serves as the driving force for crystallization. In general, Δ G ( T ) will be larger than 0 for T < T melt (that is, the crystalline phase is energetically more favourable than the liquid phase), equal to 0 at T = T melt , and smaller than 0 for T > T melt (that is, the liquid phase is more favourable than the crystalline phase). The expression for Δ G commonly used for phase change materials is the Thompson–Spaepen approximation [16] , which was also employed by Orava et al. [14] and Salinga et al. [15] : where Δ H m is the heat of fusion. In equation (1), η ( T ) denotes the viscosity, the physical quantity that limits the crystallization process counteracting the driving force and that is coupled to the atomic diffusivity through the Stokes–Einstein equation. As the molten phase change material is being cooled below the melting temperature (in the so-called super-cooled liquid state), the viscosity steadily increases with cooling, and it becomes increasingly difficult to sample all possible configurations for a given temperature. Eventually, the liquid falls out of internal equilibrium and forms a glass [17] . This process is expected to depend on the cooling rate: at slower cooling rates, the system will remain longer in internal equilibrium than for faster cooling [18] , [19] , [20] . Whether the material is in the glass state or in the super-cooled liquid state will influence the temperature dependence of the viscosity. In this article, we exploit the nanoscale dimensions and the fast thermal dynamics of a PCM cell to obtain the temperature dependence of crystal growth in both the glass and super-cooled liquid states. This also enables measurement on the melt-quenched phase directly in the environment in which the material is going to be used. Note that the interface and stress conditions will be substantially different in this case, and this could also influence the crystallization dynamics significantly [21] , [22] , [23] . In a PCM cell, a layer of crystalline phase change material is sandwiched between two electrodes. The application of a voltage pulse will result in substantial Joule heating within the PCM cell and can be used to reversibly change the phase of a nanometric volume of the phase change material to the less-ordered amorphous state and back to the more-ordered crystalline state [24] . The ‘amorphization’ process requires that the temperature within the cell be higher than the melting temperature of the phase change material. As the molten phase change material is quenched rapidly to a lower temperature, the atomic configurations are frozen into the less-ordered amorphous state [24] . The thermal dynamics of a PCM cell are fast enough to enable quench rates on the order of 10 11 Ks −1 . Our objective is to measure the crystal growth of such an amorphous state. The identification of v g ( T ) consists of four steps. In the first step, we employ isothermal experiments to directly measure the growth velocity at low temperatures. In the second step, the melting temperature, where crystal growth is zero, is estimated. In the third step, we estimate the temperature at which the growth rate is maximum. And in the fourth and final step, we obtain the overall temperature dependence of crystal growth that describes the extent of crystal growth at the amorphous–crystalline interface. For step four, the measurements from steps one to three will also serve as constraints. The experimental methodology heavily relies on the spatial and temporal evolution of temperature within the PCM cell by the application of suitable voltage signals. Measurement of growth velocity at low temperatures First, we investigate the growth velocity at low temperatures through an isothermal technique. An amorphous region is created in the PCM cell by applying a voltage pulse and thus heating a substantial part of the cell above the melting temperature, followed by quenching to the ambient temperature. The idea is to monitor the subsequent reduction of the amorphous thickness ( u a ) as a function of the ambient temperature. This approach is comparable to that presented by Salinga et al. [15] , the main differences being the manner in which the amorphous region is created and the way in which the crystal growth rate is quantified. As shown in Fig. 1a , after an amorphous region has been created, u a reduces during the time t growth until the proportionality between the electronic threshold switching voltage V th and u a is used to quantify the reduction (see Methods and Supplementary Note 1 for more details). As the melt-quenched amorphous state is in an unstable state, we need to consider the implications of structural relaxation while monitoring the reduction of u a . Because of structural relaxation, the viscosity increases with time, which according to equation (1) will cause a reduction in the growth velocity over time that has to be accounted for. 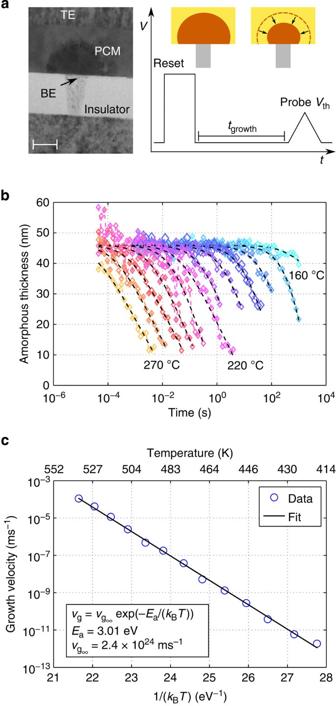Figure 1: Isothermal measurement of growth velocity. (a) Transmission electron micrograph of a ‘mushroom’ cell showing a semi-spherical amorphous dome over a heater electrode. The top electrode and bottom electrode are denoted by ‘TE’ and ‘BE’, respectively and are made of titanium nitride. Scale bar, 50 nm. The sketch of the experimental conditions shows how the amorphous dome shrinks over time until it is measured using an electrical pulse that determines the amorphous thickness via the threshold switching voltage,Vth. (b) Measured amorphous thickness as a function of time over the temperature range of 160–270 °C in steps of 10 °C. The initial amorphous thickness reduces increasingly faster for higher temperatures. Fits to the data are shown as black dashed lines. (c) The growth velocity for different temperatures determined via fitting the data displayed in (b) exhibits an Arrhenius behaviour with an activation energy of 3.01 eV. The temperatures have been corrected for the difference in temperature between the heating stage and the PCM chip. The increase of viscosity with time is well captured by [25] Figure 1: Isothermal measurement of growth velocity. ( a ) Transmission electron micrograph of a ‘mushroom’ cell showing a semi-spherical amorphous dome over a heater electrode. The top electrode and bottom electrode are denoted by ‘TE’ and ‘BE’, respectively and are made of titanium nitride. Scale bar, 50 nm. The sketch of the experimental conditions shows how the amorphous dome shrinks over time until it is measured using an electrical pulse that determines the amorphous thickness via the threshold switching voltage, V th . ( b ) Measured amorphous thickness as a function of time over the temperature range of 160–270 °C in steps of 10 °C. The initial amorphous thickness reduces increasingly faster for higher temperatures. Fits to the data are shown as black dashed lines. ( c ) The growth velocity for different temperatures determined via fitting the data displayed in ( b ) exhibits an Arrhenius behaviour with an activation energy of 3.01 eV. The temperatures have been corrected for the difference in temperature between the heating stage and the PCM chip. Full size image and from equation (1), v g ( t ) is assumed to be inversely proportional to η ( t ), leading to where is a constant and denotes the growth velocity at t =0. Then, the evolution of the amorphous thickness u a can be expressed as where denotes the initial amorphous thickness. Experimentally, the PCM cell was set to an elevated ambient temperature using a heating stage. Thereafter, amorphous regions were created in the PCM cell with an estimated of 46 nm by applying voltage pulses. The quench time is ~\n10 ns. The subsequent evolution of u a as a function of time is measured. The experiment is repeated for ambient temperatures ranging from 353 to 543 K. The results are shown in Fig. 1b together with the fitted time evolution from equations (4) and (5). From the fits, is obtained and shown in Fig. 1c . It can be seen that it follows a straight Arrhenius behaviour over the full range of temperatures, with an activation energy of 3.01 eV. This is suggestive of the fact that over this temperature range the amorphous region created is in the glass state. Besides the Arrhenius behaviour, another good indicator of the glassy nature is the structural relaxation that manifests as the temporal evolution of viscosity as well as the electronic threshold switching field. There is no indication of any saturation of this temporal evolution before crystallization as would be expected if the system approached equilibrium (super-cooled liquid). Remarkably, the Arrhenius behaviour spans eight orders of magnitude, extending all the way to ~\n540 K, far above typical, experimentally observed glass-transition temperatures in as-deposited amorphous phase change materials [26] . This transition from super-cooled liquid to the glass state occurring at very high temperatures could be due to the very fast quench rates in our experiment. Other aspects, such as being in a confined cell and the subsequent impact of stress, and other interfacial effects could also influence this behaviour [21] , [23] . Measurement of T melt Next, we present the measurement of the melting temperature T melt at which the crystallization rate becomes zero. An experiment is performed to detect the dissipated electrical power within the PCM cell during the application of voltage pulses needed to initiate melting. This measurement is repeated over a wide range of ambient temperatures, and the power needed to initiate melting is obtained as a function of the ambient temperature. The essential idea is that from this data one can predict the ambient temperature that corresponds to the limiting case of zero dissipated power, which would correspond to the melting temperature of the phase change material. In the mushroom-type PCM cell (as depicted in Fig. 2a ), finite-element simulations indicate that the maximum temperature is reached very close to the bottom electrode [27] , [28] , [29] . This is due to the significant asymmetry between the dimensions of the top and bottom electrodes. The substantially smaller bottom electrode and hence higher current density ensure that most of the electric power is dissipated within the phase change material close to the bottom electrode. This causes a rise in temperature, which will be balanced by the heat transport away from the cell. By averaging over all possible heat pathways through materials with very different thermal conductivities and geometric contributions, an average thermal resistance R th for the heat transported away can be defined. 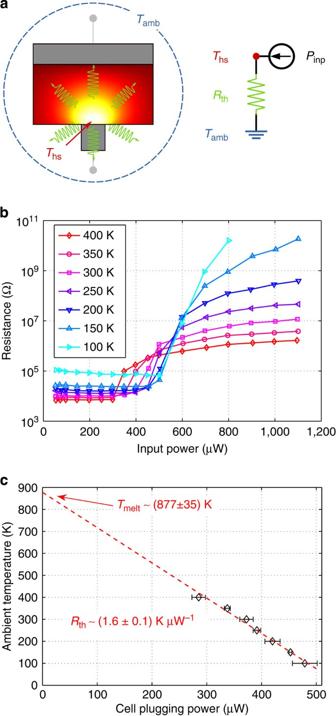Figure 2: Measurement of the melting temperature. (a) Finite-element simulation indicating the temperature distribution in a mushroom-type PCM cell upon application of a voltage pulse with power,Pinp. The temperature close to the bottom electrode is referred to as the hotspot temperature,Ths. The heat loss (indicated in green) can be modelled with an equivalent thermal resistanceRththat captures the thermal resistance of all possible heat pathways. The PCM cell is operated within an ambient temperature,Tamb. (b) After the application of the voltage pulse, the electrical resistance is measured. The resistance as a function ofPinpobtained at different ambient temperaturesTambis shown. At a certainPinp, denoted byPmelt, melting will be initiated within the PCM cell (ThsequalsTmelt) and this results in the plugging of the bottom electrode by the amorphous phase. This plugging results in a sharp increase in the resistance from the value corresponding to the fully crystalline PCM cell.Pmeltincreases with decreasingTambbecause of the higher temperature difference betweenTambandTmelt(equation (7)). (c)Pmeltas a function ofTambobtained by repeating the experiments 10 times is shown with the error bar indicating the standard deviation. Using equation (7),TmeltandRthare obtained from ordinate intercept and slope, respectively. Figure 2: Measurement of the melting temperature. ( a ) Finite-element simulation indicating the temperature distribution in a mushroom-type PCM cell upon application of a voltage pulse with power, P inp . The temperature close to the bottom electrode is referred to as the hotspot temperature, T hs . The heat loss (indicated in green) can be modelled with an equivalent thermal resistance R th that captures the thermal resistance of all possible heat pathways. The PCM cell is operated within an ambient temperature, T amb . ( b ) After the application of the voltage pulse, the electrical resistance is measured. The resistance as a function of P inp obtained at different ambient temperatures T amb is shown. At a certain P inp , denoted by P melt , melting will be initiated within the PCM cell ( T hs equals T melt ) and this results in the plugging of the bottom electrode by the amorphous phase. This plugging results in a sharp increase in the resistance from the value corresponding to the fully crystalline PCM cell. P melt increases with decreasing T amb because of the higher temperature difference between T amb and T melt (equation (7)). ( c ) P melt as a function of T amb obtained by repeating the experiments 10 times is shown with the error bar indicating the standard deviation. Using equation (7), T melt and R th are obtained from ordinate intercept and slope, respectively. Full size image If T hs is the temperature corresponding to the region just above the bottom electrode in the cell, as also shown by Boniardi et al. [30] , it is possible to write where P inp is the input power associated with the voltage pulse and T amb the ambient temperature. The low-field resistance measurement as a function of the input power provides an estimate of how the amorphous thickness evolves as a function of the dissipated power [31] . One particularly interesting point in such a map of resistance versus input power is the one that corresponds to the onset of ‘plugging’ of the bottom electrode with amorphous phase change material. At this point, the first measurable increase in the resistance of the cell will occur, and T hs will be approximately equal to the melting temperature of the phase change material. Then in steady state, the following equation holds: where P melt is the power required to reach the melting temperature at the onset of plugging. Assuming that T melt and R th remain constant, only P melt will vary with the ambient temperature. The melting temperature can therefore be obtained by extrapolation of the P melt versus T amb data. Voltage pulses of varying amplitude with a duration of 1,000 ns were applied to the cell to ensure steady-state melting, with sharp edges to prevent unwanted re-crystallization. The current that flows through the PCM cell was measured and the dissipated power calculated. The low-field electrical resistance was measured at the end of the application of each pulse, and the map between the cell resistance and the input power was obtained. The experiment was repeated at different ambient temperatures from 100 to 400 K in steps of 50 K. The map between the cell resistance and the input cell power is shown in Fig. 2b . The low-field resistance reduces with increasing T amb in both phases due to an increase in the thermally activated carriers. The ‘jump’ in resistance in each curve corresponding to P melt decreases with T amb . This experiment was repeated 10 times; the resulting experimentally measured P melt as a function of T amb is shown in Fig. 2c . The fit with equation (7) allows an estimate of the melting temperature and the effective thermal resistance from the y intercept and slope, respectively. The melting temperature was estimated to be 877 K. Moreover, the thermal resistance value of ~\n1.6 Kμ W −1 is a good measure of the thermal efficiency of the PCM cell. Interestingly, the T melt corresponding to the melt-quenched phase was found to be comparable to the T melt of the as-deposited phase of the same material measured using time-resolved X-ray diffraction (see Supplementary Note 2 ). Measurement of T cryst From equation (1), it is expected that a certain temperature value exists at which the crystallization rate is maximum, denoted by T cryst . The determination of this peak temperature will be discussed next. The experimental methodology consists of creating an amorphous region with a certain thickness within a PCM cell. Subsequently, we measure the power dissipated within the cell that results in the largest reduction of the initial amorphous thickness. This experiment is repeated over a wide range of ambient temperatures. From those data, the temperature that corresponds to the highest rate of crystallization can be obtained by extrapolating to the limiting case of zero crystallizing power, analogous to the determination of the melting temperature in the preceding section. A two-stepped voltage pulse is applied to a PCM cell, as shown in the first panel of Fig. 3b , such that the amplitude of the first part of the pulse induces substantial, steady-state melting within the PCM cell and the second part of the pulse induces re-crystallization of the amorphous region created by the application of the first part of the pulse. The crystal growth rate will mostly be determined by the interfacial temperature T int between the crystalline and amorphous phases. 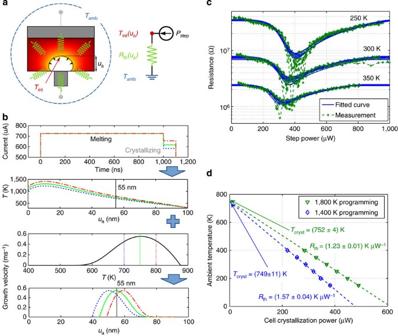Figure 3: Measurement of the temperature of maximum growth velocity. (a) Schematic illustration of the re-crystallization process during the application of a two-stepped pulse. The melting part of the pulse creates an amorphous region of thickness,ua, indicated by the black dashed line. During the application of crystallizing part of the pulse with power,Pstep, the amorphous–crystalline interface temperature reachesTint, which allows some re-crystallization to the final amorphous region shown in white. (b) Schematic illustration of three different voltage pulses applied to the PCM cell with different amplitudes in the crystallizing part. The melting part creates an amorphous region of thickness 55 nm. The differentPstepassociated with the crystallizing part results in three different temperature profiles and correspondingly three differentTint. In the case shown here, the green pulse results in achieving theTintthat corresponds to the maximum crystal growth whereas the red and blue pulses result in higher and lowerTint, respectively and this leads to lesser growth. (c) The electrical resistance as a function ofPstepis obtained at different ambient temperatures. The averaged minima of the fits denote the power at which the maximum growth velocity is reached at the interface denoted byPcryst.Pcrystincreases with reducing ambient temperature. (d)Pcrystas a function ofTambobtained by repeating the experiment 10 times is shown with the error bar indicating the s.d. Following equation (10), the temperature of maximum growth velocity,Tcrystand the equivalent thermal resistance from the interface,Rthare obtained from ordinate intercept and slope, respectively. The experiment was done for two different initial amorphous thicknesses. The rate of change of amorphous thickness can be written as Figure 3: Measurement of the temperature of maximum growth velocity. ( a ) Schematic illustration of the re-crystallization process during the application of a two-stepped pulse. The melting part of the pulse creates an amorphous region of thickness, u a , indicated by the black dashed line. During the application of crystallizing part of the pulse with power, P step , the amorphous–crystalline interface temperature reaches T int , which allows some re-crystallization to the final amorphous region shown in white. ( b ) Schematic illustration of three different voltage pulses applied to the PCM cell with different amplitudes in the crystallizing part. The melting part creates an amorphous region of thickness 55 nm. The different P step associated with the crystallizing part results in three different temperature profiles and correspondingly three different T int . In the case shown here, the green pulse results in achieving the T int that corresponds to the maximum crystal growth whereas the red and blue pulses result in higher and lower T int , respectively and this leads to lesser growth. ( c ) The electrical resistance as a function of P step is obtained at different ambient temperatures. The averaged minima of the fits denote the power at which the maximum growth velocity is reached at the interface denoted by P cryst . P cryst increases with reducing ambient temperature. ( d ) P cryst as a function of T amb obtained by repeating the experiment 10 times is shown with the error bar indicating the s.d. Following equation (10), the temperature of maximum growth velocity, T cryst and the equivalent thermal resistance from the interface, R th are obtained from ordinate intercept and slope, respectively. The experiment was done for two different initial amorphous thicknesses. Full size image A schematic illustration of the re-crystallization process during application of the two-stepped pulse is shown in Fig. 3a . The thermal model corresponding to the application of the crystallizing part of the pulse can be written as where T int ( u a ) is the temperature at the interface between the amorphous and crystalline regions and P step denotes the power dissipated during application of the crystallizing part of the pulse. R th ( u a ) is the effective thermal resistance that corresponds to the u a reached during the melting part of the pulse. Varying the amplitude of the crystallizing part of a two-stepped pulse results in different temperature distributions in the cell, as shown in the second panel of Fig. 3b . As the crystal growth rate is strongly temperature-dependent, the rate of re-crystallization will change significantly based on the temperature reached at the interface. This is depicted in Fig. 3b , which shows three different pulses that result in interfacial temperatures with different growth rates (marked as vertical lines in the third panel of Fig. 3b ). If the duration of the second part of the pulse is chosen to be small, we can ensure a small change in the amorphous thickness, making linear analysis applicable. Moreover, the maximum reduction of the amorphous thickness will be achieved when T int = T cryst . If we measure the power that corresponds to this scenario, denoted by P cryst , then equation (9) becomes By measuring the cell resistance after application of the two-stepped pulse, we can obtain a map between the cell resistance and the cell input power during the crystallizing part of the pulse. The input power at which the resistance value is the smallest will correspond to P cryst . If this experiment is repeated at varying ambient temperatures, one can obtain P cryst as a function of T amb . P cryst will reduce as T amb increases, and from equation (10), we can obtain T cryst by extrapolation. Two-stepped voltage pulses with sharp transitions of 10 ns were repeatedly applied to the PCM cell while varying the amplitude of the second step. The voltage corresponding to the melting part of the pulse (first step) was chosen to obtain a given hot-spot temperature using equation (6). In this way, we can ensure that the size of the amorphous region initially created is almost identical at all ambient temperatures ( Supplementary Note 3 ). The voltage corresponding to the crystallizing part of the pulse (second step) was chosen to vary such that it spans a relevant power range for the measurement of the crystallization rate. The melting part of the pulse had a duration of 1,000 ns, whereas the crystallizing part of the pulse was chosen to be <100 ns in duration. This ensures that the reduction in amorphous thickness due to recrystallization is small enough even if the growth velocity is maximum. After application of a pulse, the electrical resistance was measured. This experiment was then repeated 10 times at ambient temperatures ranging from 150 to 400 K in steps of 50 K for two values of the programmed hot-spot temperature, T hs corresponding to two different sizes of the amorphous region: T hs =1,400 and 1,800 K. The cell resistance curves measured as a function of P step for a programmed hot-spot temperature of 1,800 K are shown in Fig. 3c for three different ambient temperatures. The power at which the resistance is minimum, which corresponds to the P cryst at which the growth rate is maximum, was obtained using a fitting procedure, the details of which are presented in the Methods section. The values of P cryst extracted for the different ambient temperatures are presented in Fig. 3d . From this, an estimate of T cryst and an estimate of the equivalent thermal resistance corresponding to the initial amorphous thickness are obtained. There is remarkable agreement between the values for T cryst obtained in both cases, with the mean value being 750 K. It can also be seen that the effective thermal resistance reduces with increasing melting power and corresponding increase of the amorphous thickness, as expected from the temperature distribution within the mushroom-type PCM cell. Estimation of v g ( T ) Having measured the crystal growth rate at low temperatures as well as having estimated T melt and T cryst , the final objective is to obtain the overall temperature dependence of the growth velocity. For this, we expand on the idea behind the experiments presented in the section ‘Measurement of T cryst ’. We use the overall variation of u a as a function of the crystallizing power and not just the power that corresponds to the maximum reduction in u a . The objective is to find the v g ( T ) that describes the variation of u a as a function of the crystallizing power at all ambient temperatures under the constraints set by the preceding experiments. First of all, we need an accurate estimate of u a . This was obtained by measuring the current–voltage characteristic, in addition to the resistance measurements, after application of each two-stepped pulse. u a is calculated using the electrical transport model proposed by Ielmini and Zhang [32] (see Methods). For the programmed hot-spot temperature of 1,800 K, we obtained a u a estimate of ~\n55 nm for all ambient temperatures when the crystallizing step power is zero. The estimated u a as a function of P step for four different values of T amb is shown in Fig. 4a . 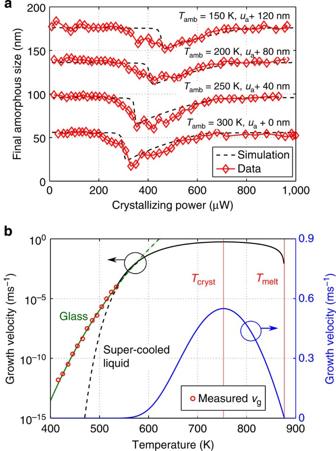Figure 4: Estimation of the overall temperature dependence of growth velocity. (a) Estimated amorphous thickness,ua, as a function of the crystallizing power corresponding to the two-stepped pulse (Pstep) obtained at different ambient temperatures. The curves are shifted vertically for clarity. Also shown is the comparison with theuaversusPsteprelationship obtained by solving equations (8) and (9) using the estimated temperature dependence of growth velocity,vg(T). (b) The estimatedvg(T) plotted in log and linear scales along with the results from the preceding sections. In the log plot, the estimatedvg(T) is depicted by solid lines (black and green). The black solid line captures the growth rate in the super-cooled liquid state, where the growth velocity is described by equation (1) and the viscosity is given by equation (11). At a temperature of 534 K,vg(T) deviates from the super-cooled liquid behaviour and follows an Arrhenius behaviour characteristic of the glass state as described by equation (13) (denoted by the green solid curve). The black dashed line indicates the extrapolation of the super-cooled liquid behaviour to lower temperatures, and the green dashed line shows the extrapolation of the Arrhenius behaviour to higher temperatures. Figure 4: Estimation of the overall temperature dependence of growth velocity. ( a ) Estimated amorphous thickness, u a , as a function of the crystallizing power corresponding to the two-stepped pulse ( P step ) obtained at different ambient temperatures. The curves are shifted vertically for clarity. Also shown is the comparison with the u a versus P step relationship obtained by solving equations (8) and (9) using the estimated temperature dependence of growth velocity, v g ( T ). ( b ) The estimated v g ( T ) plotted in log and linear scales along with the results from the preceding sections. In the log plot, the estimated v g ( T ) is depicted by solid lines (black and green). The black solid line captures the growth rate in the super-cooled liquid state, where the growth velocity is described by equation (1) and the viscosity is given by equation (11). At a temperature of 534 K, v g ( T ) deviates from the super-cooled liquid behaviour and follows an Arrhenius behaviour characteristic of the glass state as described by equation (13) (denoted by the green solid curve). The black dashed line indicates the extrapolation of the super-cooled liquid behaviour to lower temperatures, and the green dashed line shows the extrapolation of the Arrhenius behaviour to higher temperatures. Full size image Next, the differential equation (8) in combination with equation (9) was numerically solved for the time interval t step , denoting the width of the crystallizing part of the two-stepped pulse. The thermal resistance of the cell as a function of the amorphous thickness, R th ( u a ), is needed for this; it was extracted from finite-element modelling in combination with experimental measurements (see Methods and Supplementary Note 4 ). To estimate v g ( T ), a parametric model is needed. At high temperatures, v g ( T ) is assumed to follow the growth rate description associated with the super-cooled liquid state given by equation (1), where the viscosity is provided by one of the most recent and most accurate models to describe its temperature dependence [33] , namely, where η ∞ is the extrapolated infinite temperature viscosity. T g is the temperature defined to be the temperature at which viscosity equals 10 12 Pa s and m denotes the fragility given by However, below a certain transition temperature, T glass , the growth rate has to deviate from that of the super-cooled liquid state to match the measured values from the isothermal experiment presented earlier. Based on these measurements, the growth velocity is captured by an Arrhenius behaviour characteristic of the glass state given by where the activation energy E a is 3.01 eV and v g ∞ =2.4 × 10 24 ms −1 . Hence, v g ( T ) is constituted by two segments, one that corresponds to the super-cooled liquid state and the other that corresponds to the glass state. By iterating over the parameters, T g , m , η ∞ and T glass , the best estimate of v g ( T ) that fits the u a versus P step data for all four ambient temperatures was obtained. The melting temperature, T melt , entering into v g ( T ) via equation (2), was set to the measured value of 877 K Δ H m was set to 152.4 meV per atom, which is a value from literature for as-deposited Ge 2 Sb 2 Te 5 (ref. 34 ). Moreover, v g ( T ) was constrained to have a maximum value at T cryst based on the results from the preceding section. The parameters λ and r atom in equation (1) were chosen to be 0.299 and 0.1365, nm, respectively, and R hyd = r atom . The fit parameters T g , m , η ∞ and T glass were obtained to be 472 K, 140, 0.012 Pa s and 534 K, respectively. The fits to the experimental data are shown in Fig. 4a . The fits are particularly good at crystallization powers above P cryst . In this regime, the crystallization process is self-limiting. The temperature at the interface is higher than T cryst and a shrinkage in amorphous thickness leads to decreasing values of v g ( Fig. 3b ). For crystallization powers below P cryst , the simulation exhibits a sharp drop in the amorphous thickness because the re-crystallization is self-accelerating once the interface temperature falls below T cryst and a reduction in u a will lead to even higher re-crystallization speed. In the experiment, this is less pronounced, possibly because of the averaging over the interface temperatures. In addition, the self-acceleration could amplify the small variations in the programmed u a , thus making the data more noisy. The estimated v g ( T ) along with the results from the preceding sections are shown in Fig. 4b . The blue solid line shows v g ( T ) in the linear scale, whereas the black and green solid lines describe v g ( T ) in the log scale. The black line (solid and dashed) corresponds to the super-cooled liquid state, where the growth velocity is described by equation (1) and the viscosity is given by equation (11). The fragility, m , which was one of the fit parameters and found to have a high value of 140, corresponds to the super-cooled liquid state. However, even at a rather high temperature of 534 K, the glass state is formed, possibly owing to the ultra-fast quench rates. Below this temperature, the growth velocity deviates from that of the super-cooled liquid state and follows an Arrhenius behaviour as described by equation (13) (denoted by the green solid line). The green dashed line depicts the extrapolation of the Arrhenius behaviour to higher temperatures, and the black dashed line shows the extrapolation of the super-cooled liquid behaviour to lower temperatures. It can be seen that the crystallization rate is significantly higher for the glass state than for the corresponding super-cooled liquid state. However, as pointed out earlier, there is also a temporal component to the crystallization rate of the unstable glass state, whereby the growth velocity decreases with increasing time and thus possibly approaches the growth rate corresponding to the super-cooled liquid state over time. Using the isothermal method, we were able to measure the growth velocity of the melt-quenched phase change material up to ~\n 540K, which is about as high as the highest reported temperature to which a phase change material has been measured so far [15] . In doped Ge 2 Sb 2 Te 5 , we observed an Arrhenius behaviour over eight orders of magnitude in growth velocity. This remarkable result confirms the wide range of singly activated behaviour previously observed in a very different phase change material, namely, Ag- and In-doped Sb 2 Te (ref. 15 ). As Δ G <0.18 eV is much lower than E a ≈3 eV in the glass state below 534 K, the observed Arrhenius behaviour shows that also in the melt-quenched state in memory cells the activation energy for diffusion controls the temperature dependence of the growth velocity [34] , [35] . It is also worth noting that we do not find sufficient evidence of a breakdown of the Stokes–Einstein relation between diffusivity and viscosity, which would introduce an exponent ξ <1 for the viscosity term η in equation (1) [36] ( Supplementary Note 5 ). The high activation energy for crystallization in the glass state explains the ability of these materials to crystallize on the nanosecond timescale at elevated temperatures while being able to retain the amorphous state for several years at room temperature. As can be seen in Fig. 4b , the high activation energy together with the ultra-fast quench rate leads to a smooth glass transition at very high temperatures, which might be the reason why so far no clear discontinuity in activation energy has been observed in the literature, in contrast to other fragile glasses such as polymers. The analysis of the isothermal measurement also nicely demonstrates the complexity of the behaviour of the glass state, and that it is crucial to consider relaxation during long-term experiments as it influences both viscosity and electrical transport. The ultra-fast quench rates mean that the glass state formed in a PCM cell is far from thermal equilibrium. This is unlike samples produced by sputter deposition. Hence, one of the biggest blessings (the fast speed of the materials) also leads to the biggest curse of the technology, namely, the structural relaxation towards the equilibrium that is observed in our work and in literature as drift in growth rate, threshold voltage and resistance [37] . In particular, the last is a significant challenge in realizing multi-level storage [31] , [38] . Another consequence of this finding is that the simple extrapolation typically done for evaluating the retention time of stored information [39] , [40] needs to be corrected for the temporal slow-down of crystal growth upon drift. Despite the tremendous increase of the temperature range over which recent studies have investigated the crystal growth velocity, still only the left side of T cryst had been probed [14] , [15] . Going beyond those studies, we also probed the dynamic behaviour of the melt-quenched material around and above the maximum of the growth velocity all the way up to the melting temperature. From a technological standpoint, the information about the melting temperature and the temperature of highest growth velocity is very important for the performance evaluation of a material directly measured within a cell. Apart from the cell design, the melting temperature is ultimately the limiting factor for the energy efficiency, and the temperature of maximum growth influences the data retention and the vulnerability to thermal disturbance. As those decisive material properties are measured directly in a memory cell, it is also possible to measure those quantities as a function of cycling and drift. Especially the change of those performance factors with cycling is critical because it has been shown that the material composition within a cell may change during the lifetime of operation, for example, because of electromigration [41] , [42] . To summarize, we have obtained, for the first time, a comprehensive picture of the temperature dependence of the crystal growth of melt-quenched phase change materials. It is expected that these results and methodology will have a significant impact on fundamental research on the phase change mechanism as well as super-cooled liquids and glasses in general. The technological relevance stems from the central role played by crystal growth in phase change-based electronic devices, influencing properties such as the speed of operation, energy consumption and retention of a certain phase configuration. Moreover, the fact that the measurements can be performed within the confines of nanoscale devices in which the material is going to be used opens up several new avenues for future work. PCM cells The mushroom-type PCM cells used in the experiments were fabricated in the 90-nm technology node with the bottom electrode created via sub-lithographic key-hole process [43] . The phase change material is doped Ge 2 Sb 2 Te 5 . The dopant is primarily intended to enhance the endurance of the PCM cell [44] . All experiments were conducted on PCM cells that had been heavily cycled. The bottom electrode has a radius of ~\n20 nm and a length of ~\n65 nm. The phase change material has a thickness of 100 nm and extends to the top electrode, whose radius is ~\n100 nm. Experimental setup Most of the measurements were done on a JANIS ST-500-2-UHT cryogenic probing station that operates from 77 to 400 K and offers a temperature stability of <50 mK. The cryostat is cooled by using liquid nitrogen as a cryogen. Two heaters with powers of 50 and 25 W and at different positions in the chamber allow temperature control. The temperature is measured at four points inside the chamber by calibrated Lakeshore Si DT-670B-CU-HT diodes with an accuracy of <0.5 K. Temperature was regulated using a Lakeshore 336 Automatic Temperature Controller. To thermally isolate the sample, a radiation shield is fixed above the sample mount and thermally connected to the nitrogen out flux. To avoid heat exchange via convection and water condensation at low temperatures, the experiments were done under vacuum (average pressure of 10 −5 mBar). The chamber has six ports. Only one of them was used to connect a high-frequency Cascade Microtech Dual-Z probe. The high-frequency probe is connected with cooling braids to the Cu chuck to guarantee that the sample and the probe are at the same temperature. The sample is fixed on the Cu sample mount inside the vacuum chamber by a metal clip. A Keithley 2400 SMU was used for DC voltage or current outputs and the measurement of the corresponding current or voltage at the sample. An Agilent 81150A Pulse Function Arbitrary Generator was used for AC voltage outputs (cell switching) and a Tektronix TDS3054B oscilloscope for AC voltage and current measurements. Mechanical relays were used to switch between AC and DC measurements. The cell resistance was measured at a constant read voltage of 0.2 V and the current–voltage ( I – V ) characteristics were measured using the current output mode of the SMU from 1 nA to 1 μA. For the isothermal measurements, identical probe-head and electronics were used. However, to achieve higher temperatures, the sample was mounted on an invar block with two embedded Tungsten heaters. The temperature was measured using a thermocouple inserted into the invar block and controlled via a Eurotherm temperature controller. The temperature on top of the PCM chip was further calibrated using an Omega silicon diode sensor. The threshold switching voltage was determined by applying a triangular voltage signal of 4-μs duration. Finite-element simulations Simulations using the finite-element method have been performed using Comsol 4.3b in 2D-axial symmetry using the built-in Joule heating model. The mushroom-type geometry of the device extracted from scanning electron microscope images was rebuilt. The thermal conductivity of the electrode material (TiN), the insulator (SiO 2 ) and the phase change material was chosen to be 12 Wm −1 K −1 , 1.4 Wm −1 K −1 and 0.5 Wm −1 K −1 , respectively. The electrical conductivity of TiN was chosen to be 3.8 × 10 5 Sm −1 and SiO 2 was assumed to be a perfect insulator. The electrical conductivity of the phase change material was determined from the I – V measurements to be described as a function of the electric field. The conductivity rises roughly exponentially from 10 4 Sm −1 at low fields to 5 × 10 5 Sm −1 at 55 V μm −1 ( Supplementary Note 4 ). The boundaries of the model in the SiO 2 domains were chosen to be thermally and electrically insulating. The boundaries for the top and bottom electrodes were set to be at constant temperature, and a voltage potential was applied. At the interface between TiN and the phase change material, a thermal boundary resistance of 20 m 2 K GW −1 was implemented. Estimation of u a from V th A fast estimate of the amorphous thickness can be obtained as follows. The threshold switching voltage is linked to the amorphous thickness by [22] E th denotes the threshold switching field at which the electronic threshold switching takes place. At this critical field, the resistance of the PCM cell drops to a substantially lower value, resulting in a sharp increase in the current [45] , [46] . However, E th ( t ) itself undergoes an evolution with time owing to the structural relaxation of the amorphous phase. A good empirical model describing such a temporal evolution is given by [47] where ν E is the drift coefficient of the threshold field and is the threshold field at t = t 0 . A fixed value of ν E was assumed for all temperatures and can be estimated from experiments conducted at low ambient temperatures at which the crystal growth rate is negligible. The threshold switching voltage data V th ( t ) (shown in Supplementary Note 1 ) was then fitted to equation (14) in conjunction with equations (15) and (5) with , and Q as fitting parameters. The resulting u a ( t ) and are shown in Fig. 1b,c , respectively. Fitting procedure for resistance versus P step curves To obtain the power at which the resistance is minimum in the resistance versus P step data, the experimental data was fitted to a parametric R ( P step ) curve. This is done to minimize the impact of noise. The parametric R ( P step ) curve was in turn based on a characteristic u a ( P step ) curve obtained using the simulations described in Section Estimation of v g ( T ) and is given by where x s , x o , y s and y o were the fitting parameters. The scaling and offsetting using these parameters is necessary because the exact relationship between the resistance and u a in a mushroom cell geometry is not exactly linear especially at higher u a values, owing to resistance spreading in the mushroom geometry [31] . However, this does not pose a significant problem as we are only interested in obtaining the P step value at which the minimum resistance value is measured. Estimate of u a from sub-threshold I – V measurements To estimate the amorphous thickness, I – V measurements were made. The low-field region of the I – V curve before threshold switching is fitted with the model for sub-threshold electrical transport by Ielmini and Zhang [32] where q denotes the elementary charge. The fitted parameters were r E , an effective bottom electrode radius introduced to accurately model the resistance spreading in the mushroom cell design, and the effective amorphous thickness u a (refs 31 , 48 ). The other parameters were left constant; τ 0 =10 −14 s, Δ z =6.9 nm, ε a =0.34 eV and T = T amb . Estimation of R th ( u a ) Finite-element modelling in combination with experimental techniques can be used to estimate R th ( u a ). The two-stepped pulse approach employed to measure T cryst can also be used to obtain R th ( u a ). At a fixed ambient temperature, two-stepped pulses are applied and P cryst is measured. These experiments are repeated by varying the amplitude of the melting part of the pulse across a wide range, thus changing the size of the initial amorphous region created within the PCM cell. From the resulting relationship between the initial amorphous thickness and the corresponding P cryst measurements, one can estimate R th ( u a ) using equation (10) and the estimated T cryst =750 K. There is remarkable agreement between this estimate and that obtained from FEM ( Supplementary Note 4 ). Given the uncertainties associated with the effective thermal resistance surrounding the memory cell, the R th ( u a ) obtained through FEM is scaled down by a factor of 1.15 to match the experimental measurements more accurately. This is equivalent to introducing a constant heat flux boundary condition in the FEM simulation. How to cite this article: Sebastian, A. et al. Crystal growth within a phase change memory cell. Nat. Commun. 5:4314 doi: 10.1038/ncomms5314 (2014).